Impaired thermogenesis and adipose tissue development in mice with fat-specific disruption of insulin and IGF-1 signalling Insulin and insulin-like growth factor 1 (IGF-1) have important roles in adipocyte differentiation, glucose tolerance and insulin sensitivity. Here to assess how these pathways can compensate for each other, we created mice with a double tissue-specific knockout of insulin and IGF-1 receptors to eliminate all insulin/IGF-1 signalling in fat. These FIGIRKO mice had markedly decreased white and brown fat mass and were completely resistant to high fat diet-induced obesity and age- and high fat diet-induced glucose intolerance. Energy expenditure was increased in FIGIRKO mice despite a >85% reduction in brown fat mass. However, FIGIRKO mice were unable to maintain body temperature when placed at 4 °C. Brown fat activity was markedly decreased in FIGIRKO mice but was responsive to β3-receptor stimulation. Thus, insulin/IGF-1 signalling has a crucial role in the control of brown and white fat development, and, when disrupted, leads to defective thermogenesis and a paradoxical increase in basal metabolic rate. Obesity, that is, excess body fat, is associated with the development of metabolic disorders such as type 2 diabetes, hyperlipidemia and cardiovascular disease and fatty liver [1] . Obesity results from an imbalance between energy expenditure and energy intake resulting in a positive energy balance. White adipose tissue (WAT) is the main energy storage organ in the body, whereas brown adipose tissue (BAT) is an essential component of energy expenditure by dissipating energy as heat through uncoupled respiration mediated by uncoupling protein 1 (UCP1). While BAT persists after birth in small mammals, its presence in humans was thought to be limited to newborns. However, recent studies using positron emission tomography (PET) imaging have shown that BAT is present in adult humans and is functionally active [2] , [3] , [4] , [5] , [6] . Both white and brown adipose tissue development and expansion occur through differentiation of preadipocytes into adipocytes, as well as storage and mobilization of lipids. Many paracrine and endocrine factors control adipose tissue development [7] . Among them, insulin and IGF-1 have an essential role in stimulating cell proliferation, differentiation and lipid accumulation [8] , [9] . Both insulin receptors (IR) and IGF-1 receptors (IGF1R) are present in preadipocytes and adipocytes, with more IGF1R in preadipocytes and more IR in adipocytes [10] , [11] , [12] . While insulin and IGF-1 bind preferentially to their cognate receptors, we have shown that IR and IGF1R can act as identical portals in the regulation of gene expression and adipocyte differentiation in preadipocytes [12] . Thus, when the IR [13] , [14] or IGF1R [15] is inactivated in adipose tissue, the other member of this receptor family can take over part or all of its functions. In the present study, we have investigated the role of insulin and IGF-1 signalling in adipose tissue by creating mice lacking the IR and IGF1R in both white and brown adipose tissues by gene targeting using a Cre recombinase driven by the adipose-specific aP2 promoter. We show that Fat-specific IGF1R and IR KO (FIGIRKO) mice are resistant to age-associated and diet-induced obesity and the associated glucose intolerance. Even more striking is the almost complete absence of BAT and dramatic cold sensitivity in these mice. Nonetheless, these mice exhibit increased basal energy expenditure. Thus, insulin and IGF-1 signalling have a crucial role in controlling white and brown fat development, adipocyte metabolism and thermogenesis. FIGIRKO mice show reduced white and brown adipose tissues To investigate the overlapping signalling created by insulin and IGF-1, we created mice with a combined tissue-specific knockout of the insulin and IGF-1 receptors (IR/IGF1R) in fat by breeding mice with IR and IGF1R floxed alleles with mice carrying an aP2 promoter-Cre transgene. On normal chow, body weight of male FIGIRKO mice was decreased by 16% at 4 weeks, and this increased to a 42% reduction by 1 year of age ( Fig. 1a ). Epididymal and inguinal fat pad weights at 4 months were decreased by 24% and 53%, respectively ( Fig. 1b ). Even more striking was the >85% reduction in BAT ( Fig. 1b ). Weights of other tissues were unchanged ( Supplementary Fig. S1a ). There was no difference in cell size in the perigonadal or subcutaneous WAT between FIGIRKO and control mice, indicating that the decrease in fat mass was due to fewer, not smaller, white adipocytes ( Fig. 1c,d ). On the other hand, there was a reduction in lipid content in BAT from FIGIRKO mice ( Fig. 1c ) and a 17.2% decrease in cell diameter, indicating a decrease in both cell number and cell size in this depot. Lean mass was decreased by 10% in FIGIRKO mice, but slightly increased when normalized to total body weight, indicating that the decrease in body weight observed in FIGIRKO mice was mostly attributed to a decrease in fat mass ( Supplementary Fig. S1b ). Skeletal muscle weights were not different between control and FIGIRKO mice ( Supplementary Fig. S1c ), but femur length was decreased in FIGIRKO mice by 2–6% suggesting a mild growth defect ( Supplementary Fig. S1d ). White adipose tissue at 6 weeks old was reduced by ~20% in FIGIRKO mice, whereas interscapular BAT was decreased by 84% ( Supplementary Fig. S2a,b ). IR and IGF1R messenger RNA levels in the remaining WAT and BAT and isolated WAT adipocytes of FIGIRKO mice were decreased 30–60% compared with control, with no change in other tissues ( Supplementary Fig. S3 ). 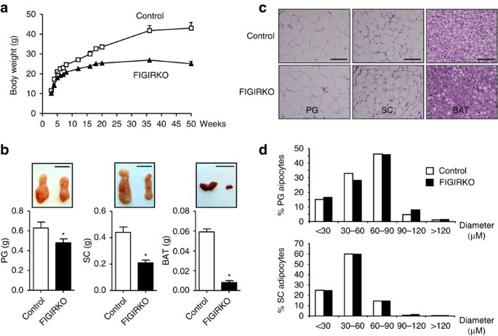Figure 1: FIGIRKO mice have reduced adiposity. (a) Body weight of male control and FIGIRKO mice fed a chow diet. Results are mean±s.e.m. of 8–15 animals/group. (b) Lower panels show perigonadal (PG), inguinal subcutaneous (SC), and brown adipose tissue (BAT) depot weights in 4 month old control and FIGIRKO male mice fed a chow diet. Results are mean±s.e.m. of 16–18 animals/group. Upper panels show representative fat pads. Scale bar=1 cm. (c) Hematoxylin and eosin stained sections of adipose tissues from male control and FIGIRKO at 4 months of age on a chow diet. Scale bar=100 μm. (d) Diameter distribution of isolated PG and SC adipocytes from 4 month old control and FIGIRKO male mice. Data represent the distribution from ~4,000 adipocytes from 4 control and 4 FIGIRKO mice. Statistical significance assessed by two-tailed Student'st-test, *P<0.05. Figure 1: FIGIRKO mice have reduced adiposity. ( a ) Body weight of male control and FIGIRKO mice fed a chow diet. Results are mean±s.e.m. of 8–15 animals/group. ( b ) Lower panels show perigonadal (PG), inguinal subcutaneous (SC), and brown adipose tissue (BAT) depot weights in 4 month old control and FIGIRKO male mice fed a chow diet. Results are mean±s.e.m. of 16–18 animals/group. Upper panels show representative fat pads. Scale bar=1 cm. ( c ) Hematoxylin and eosin stained sections of adipose tissues from male control and FIGIRKO at 4 months of age on a chow diet. Scale bar=100 μm. ( d ) Diameter distribution of isolated PG and SC adipocytes from 4 month old control and FIGIRKO male mice. Data represent the distribution from ~4,000 adipocytes from 4 control and 4 FIGIRKO mice. Statistical significance assessed by two-tailed Student's t -test, * P <0.05. Full size image FIGIRKO mice are protected against glucose intolerance In 4-month old mice, fed and fasted glucose and insulin levels ( Supplementary Fig, S4a,b ), and glucose tolerance ( Supplementary Fig. S4c ) were all similar between control and FIGIRKO mice. However, by 1 year of age fasting glucose ( Fig. 2a ) and glucose tolerance was better in FIGIRKO mice than controls ( Fig. 2b ). This occurred without any difference in insulin sensitivity as measured by insulin tolerance test ( Fig. 2c ) or glucose-stimulated insulin secretion ( Fig. 2d ). However, the glucose infusion rate required to maintain euglycemia during a hyperinsulinemic–euglycemic clamp was 25% higher in FIGIRKO than in controls, indicating an increase in insulin sensitivity ( Fig. 2e ). Insulin-stimulated whole-body glucose disposal was also increased by 51% in FIGIRKO mice; this was paralleled by an increase in basal endogenous glucose production ( Fig. 2e ). Insulin-stimulated glucose uptake assessed during the clamp using 14 C-2-deoxyglucose was decreased by 50% in white adipose tissue from FIGIRKO mice, but increased by 1.6–2.3-fold in skeletal muscle ( Fig. 2f ) indicating that the better glucose tolerance of FIGIRKO mice is due to increased glucose uptake in muscle. 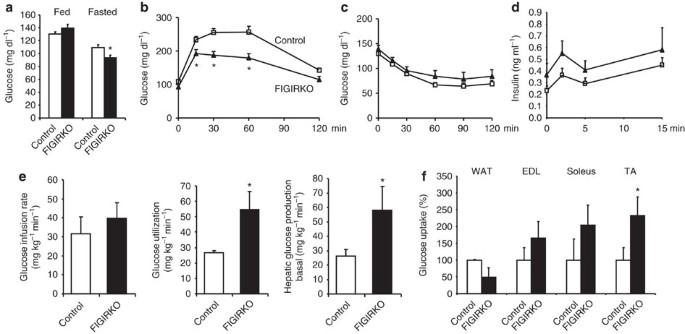Figure 2: FIGIRKO mice are protected against age-associated glucose intolerance. (a) Fed and fasted blood glucose levels in 1 year old control and FIGIRKO male mice. Results are mean±s.e.m. of 7–8 animals/group. (b) Intraperitoneal glucose tolerance test and (c) Insulin tolerance test performed in 1 year old control and FIGIRKO male mice. Results are mean±s.e.m. of 7–8 animals/group. (d) First phase insulin secretion in 1 year old male control and FIGIRKO mice. Results are mean±s.e.m. of 12 animals/group. (e) Glucose infusion rate, glucose utilization, and hepatic glucose production in the basal state, were measured during an hyperinsulinemic-euglycemic clamp. Results are mean±s.e.m. of 4 control and 5 FIGIRKO mice. (f) Insulin-stimulated14C-2-deoxyglucose uptake was assessed in perigonadal WAT, extensor digitorum longus (EDL), soleus and tibialis anterior (TA) skeletal muscles, during the final 45 min of the hyperinsulinemic-euglycemic clamp. Results are mean±s.e.m. of 4 control and 5 FIGIRKO mice. Statistical significance assessed by two-tailed Student'st-test, *P<0.05. Figure 2: FIGIRKO mice are protected against age-associated glucose intolerance. ( a ) Fed and fasted blood glucose levels in 1 year old control and FIGIRKO male mice. Results are mean±s.e.m. of 7–8 animals/group. ( b ) Intraperitoneal glucose tolerance test and ( c ) Insulin tolerance test performed in 1 year old control and FIGIRKO male mice. Results are mean±s.e.m. of 7–8 animals/group. ( d ) First phase insulin secretion in 1 year old male control and FIGIRKO mice. Results are mean±s.e.m. of 12 animals/group. ( e ) Glucose infusion rate, glucose utilization, and hepatic glucose production in the basal state, were measured during an hyperinsulinemic-euglycemic clamp. Results are mean±s.e.m. of 4 control and 5 FIGIRKO mice. ( f ) Insulin-stimulated 14 C-2-deoxyglucose uptake was assessed in perigonadal WAT, extensor digitorum longus (EDL), soleus and tibialis anterior (TA) skeletal muscles, during the final 45 min of the hyperinsulinemic-euglycemic clamp. Results are mean±s.e.m. of 4 control and 5 FIGIRKO mice. Statistical significance assessed by two-tailed Student's t -test, * P <0.05. Full size image FIGIRKO mice are protected against HFD-induced obesity When challenged with a high fat diet (HFD) for 4 months, control mice rapidly developed obesity with a 75% increase in body weight, while FIGIRKO mice were completely protected from HFD-induced weight gain ( Fig. 3a ). Accordingly, perigonadal and inguinal adipose tissues in FIGIRKO mice were markedly reduced to 28 and 8% of those in control mice after the HFD ( Fig. 3b ). Adipocyte cell size was again not different between control and FIGIRKO mice indicating that FIGIRKO mice are protected from obesity by having reduced adipocyte number. BAT mass in HFD-fed FIGIRKO mice was also reduced by 83% when compared with controls and showed reduced lipid content ( Fig. 3b ). 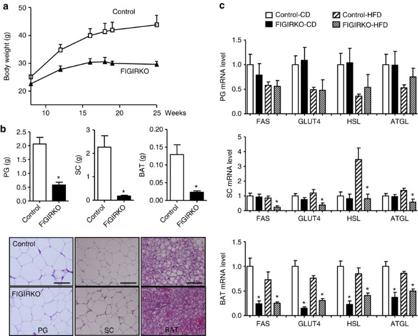Figure 3: FIGIRKO mice display resistance to HFD-induced obesity and glucose intolerance. (a) Body weight of control and FIGIRKO mice fed a HFD for 16 weeks. Results are mean±s.e.m. of 6 animals/group. (b) Adipose tissue weights (upper panel) and representative hematoxylin and eosin stained sections (lower panel) from perigonadal (PG), inguinal subcutaneous (SC), and brown adipose tissue (BAT) from 6 month old control and FIGIRKO male mice fed a HFD for 4 months. Results are mean±s.e.m. of 6 animals/group. Scale bar=100 μm (c)Fas,Glut4, HSLandATGLmRNA abundance was measured by real time PCR in perigonadal (PG), subcutaneous (SC), and brown (BAT) adipose tissues in male control and FIGIRKO mice fed either a chow diet (CD) or HFD. Results are mean±s.e.m. of 6 animals/group. Statistical significance assessed by two-tailed Student'st-test, *P<0.05. Figure 3: FIGIRKO mice display resistance to HFD-induced obesity and glucose intolerance. ( a ) Body weight of control and FIGIRKO mice fed a HFD for 16 weeks. Results are mean±s.e.m. of 6 animals/group. ( b ) Adipose tissue weights (upper panel) and representative hematoxylin and eosin stained sections (lower panel) from perigonadal (PG), inguinal subcutaneous (SC), and brown adipose tissue (BAT) from 6 month old control and FIGIRKO male mice fed a HFD for 4 months. Results are mean±s.e.m. of 6 animals/group. Scale bar=100 μm ( c ) Fas , Glut4, HSL and ATGL mRNA abundance was measured by real time PCR in perigonadal (PG), subcutaneous (SC), and brown (BAT) adipose tissues in male control and FIGIRKO mice fed either a chow diet (CD) or HFD. Results are mean±s.e.m. of 6 animals/group. Statistical significance assessed by two-tailed Student's t -test, * P <0.05. Full size image Adipocyte lipid content reflects a balance between synthesis, which is dependent on glucose uptake by glucose transporter 4 (GLUT4) and fatty acid synthase (FAS), and triglyceride breakdown, dependent on hormone sensitive lipase (HSL) and adipocyte triglyceride lipase (ATGL). In perigonadal fat, there was no difference in FAS, GLUT4, HSL or ATGL expression between control and FIGIRKO mice fed either a chow or HFD ( Fig. 3c ). There was also no difference in expression of these genes in subcutaneous adipose tissue fed a chow diet. However, there were 58–76% reductions of FAS, GLUT4, HSL and ATGL in subcutaneous fat from HFD-fed FIGIRKO mice compared with control. FAS, GLUT4, HSL and ATGL were also decreased by 42–85% in BAT from FIGIRKO mice on either chow or HFD ( Fig. 3c ). Consistent with the difference in weight gain, glucose tolerance worsened in control mice on HFD, but remained unchanged in FIGIRKO mice ( Fig. 4a ). This occurred without improvement in insulin sensitivity as measured by insulin tolerance test ( Fig. 4b ) or difference in glucose-stimulated insulin secretion ( Fig. 4c ). Random-fed insulin levels, however, were elevated sixfold in FIGIRKO mice after HFD compared with controls, possibly contributing to the improved glucose tolerance ( Table 1 ). Circulating levels of adiponectin, leptin and resistin were decreased by 42, 60 and 65% in FIGIRKO mice compared with control mice ( Table 1 ), consistent with the reduced expression of these genes in perigonadal and subcutaneous adipose ( Supplementary Fig. S5a ). 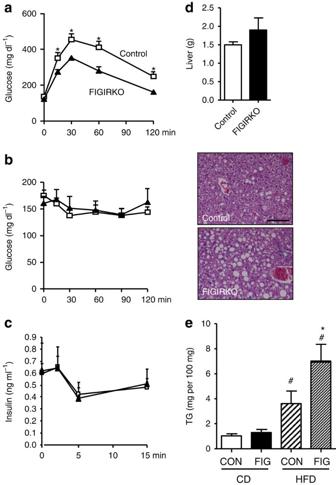Figure 4: FIGIRKO mice display resistance to HFD-induced glucose intolerance. (a) Intraperitoneal glucose tolerance, (b) insulin tolerance and (c) glucose stimulated insulin secretion tests were performed in 6 month old control and FIGIRKO male mice fed a HFD for 4 months. Results are mean±s.e.m. of 6 animals/group. (d) Liver weight (upper panel) and representative hematoxylin and eosin stained section (lower panels) from 6 month old male control and FIGIRKO mice fed a HFD for 4 months. Results are mean±s.e.m. of 6 animals/group. Scale bar=100 μm. (e) Liver triglyceride content in 6 month old male control and FIGIRKO mice fed either a chow diet (CD) or a HFD. Statistical significance assessed by two-tailed Student'st-test, *P<0.05 between control and FIGIRKO mice, #P<0.05 between CD and HFD. Figure 4: FIGIRKO mice display resistance to HFD-induced glucose intolerance. ( a ) Intraperitoneal glucose tolerance, ( b ) insulin tolerance and ( c ) glucose stimulated insulin secretion tests were performed in 6 month old control and FIGIRKO male mice fed a HFD for 4 months. Results are mean±s.e.m. of 6 animals/group. ( d ) Liver weight (upper panel) and representative hematoxylin and eosin stained section (lower panels) from 6 month old male control and FIGIRKO mice fed a HFD for 4 months. Results are mean±s.e.m. of 6 animals/group. Scale bar=100 μm. ( e ) Liver triglyceride content in 6 month old male control and FIGIRKO mice fed either a chow diet (CD) or a HFD. Statistical significance assessed by two-tailed Student's t -test, * P <0.05 between control and FIGIRKO mice, # P <0.05 between CD and HFD. Full size image Table 1 Serum parameters in chow diet or HFD-fed control and FIGIRKO mice. Full size table Obesity is often associated with hepatic steatosis. Analysis of livers from control mice on HFD revealed a 3.5-fold increase in lipid content compared with mice fed regular chow (1.03±0.17 versus 3.61±0.99 mg triglyceride per 100 mg liver). Livers from FIGIRKO mice on HFD were 20% heavier and accumulated 1.9 times more lipid than control mice ( Fig. 4d,e ). Serum triglyceride and free fatty acid levels also trended to be elevated in FIGIRKO mice on HFD, whereas cholesterol levels and circulating levels of TNFα, IL6 and PAI-1were similar ( Table 1 ). As expected, HFD resulted in increases in inflammatory markers (TNFα, MCP1 and F4/80) in both perigonadal and subcutaneous WAT of control mice. Interestingly, there was a similar increase in expression of these genes in FIGIRKO adipose tissue ( Supplementary Fig. S5b ). Thus, FIGIRKO mice on HFD develop inflammatory changes in adipose tissues compared to those of control despite the much smaller fat pad size. Increased energy expenditure in FIGIRKO mice Alterations in body weight are the balance between energy intake and energy expenditure. Food intake was similar between control and FIGIRKO mice fed either chow or HFD, suggesting that the reduction in adipose mass was due to increased energy expenditure ( Fig. 5a ). Indeed, oxygen consumption rates assessed by indirect calorimetry revealed a 15% increase in VO 2 per gram of lean body weight in FIGIRKO mice on a chow diet ( Supplementary Fig. S4d ). This occurred with no change in spontaneous activity ( Fig. 5b ). Indirect calorimetry performed in a separate cohort of FIGIRKO mice, fed a HFD from 6-to-10 months of age, confirmed a complete resistance to diet-induced obesity ( Fig. 5c ; Supplementary Fig. S6a,b ). Energy expenditure was again increased in FIGIRKO mice compared with control mice by 13–14% during the dark cycle and 7–8% during the light cycle on standard chow and HFD ( Fig. 5d ), with no difference in respiratory exchange ratio between control and FIGIRKO mice ( Fig. 5e ). Together, these results indicate that the decreased fat mass observed in FIGIRKO mice was due to a combination of a decrease in the number of adipocytes and an increase in energy expenditure. 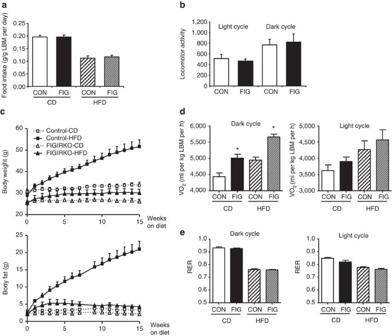Figure 5: Increased energy expenditure in FIGIRKO mice. (a) Daily food intake was measured in chow diet (CD) or HFD-fed control and FIGIRKO male mice. Mice were housed individually and food weight was measured 3 times a week for 2 consecutive weeks. For each mouse daily food intake was averaged and results are mean±s.e.m. of 6–8 animals/group. (b) Spontaneous activity was measured in control and FIGIRKO male mice fed a chow diet during 48 h. Results are mean±s.e.m. of 12 animals/group. (c) Body weight and body fat content assessed by nuclear magnetic resonance were measured weekly in 6 month old control and FIGIRKO male mice fed a chow diet or HFD for another 4 months. Results are mean±s.e.m. of 6 animals/group. (d) Oxygen consumption (VO2) and (e) respiratory exchange ration (RER) were analysed by indirect calorimetry in 10 month old control and FIGIRKO male mice fed a chow diet or a HFD for 4 months. Results are mean±s.e.m. of 6 animals/group. Dark phase is the 12h period of day during which the lights were off. Statistical significance assessed by two-tailed Student'st-test, *P<0.05. Figure 5: Increased energy expenditure in FIGIRKO mice. ( a ) Daily food intake was measured in chow diet (CD) or HFD-fed control and FIGIRKO male mice. Mice were housed individually and food weight was measured 3 times a week for 2 consecutive weeks. For each mouse daily food intake was averaged and results are mean±s.e.m. of 6–8 animals/group. ( b ) Spontaneous activity was measured in control and FIGIRKO male mice fed a chow diet during 48 h. Results are mean±s.e.m. of 12 animals/group. ( c ) Body weight and body fat content assessed by nuclear magnetic resonance were measured weekly in 6 month old control and FIGIRKO male mice fed a chow diet or HFD for another 4 months. Results are mean±s.e.m. of 6 animals/group. ( d ) Oxygen consumption (VO 2 ) and ( e ) respiratory exchange ration (RER) were analysed by indirect calorimetry in 10 month old control and FIGIRKO male mice fed a chow diet or a HFD for 4 months. Results are mean±s.e.m. of 6 animals/group. Dark phase is the 12h period of day during which the lights were off. Statistical significance assessed by two-tailed Student's t -test, * P <0.05. Full size image Decreased adipocyte differentiation in FIGIRKO mice and cells Adipocyte differentiation depends on the regulation of a transcriptional regulatory cascade involving PPARγ and proteins from the C/EBP family. In perigonadal fat, expression of C/EBPα and C/EBPβ, as well as the adipocyte marker aP2, was unchanged in FIGIRKO mice compared with controls on both chow and HFD, whereas PPARγ expression was reduced by ~40% in fat of HFD-fed FIGIRKO mice. In subcutaneous fat, PPARγ, C/EBPα, C/EBPβ and aP2 were all decreased 20 to 70% in FIGIRKO mice fed either chow or HFD ( Supplementary Fig. S5c ). For BAT, the decrease in these adipocyte differentiation genes was even more pronounced, with all four genes downregulated 20 to 90% in chow diet or HFD-fed FIGIRKO mice ( Fig. 6a ). 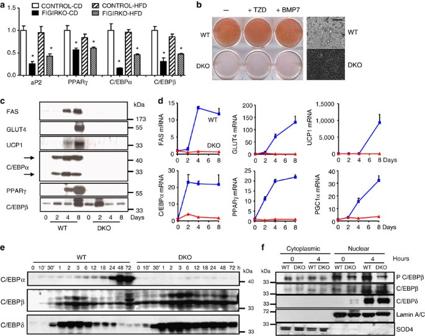Figure 6: Adipocyte differentiation is impaired in DKO brown preadipocytes. (a)aP2, PPARγ, C/EBPα andC/EBPβ mRNA abundance was measured by real time PCR in BAT from control and FIGIRKO male mice fed either a chow or a HFD. Results are mean±s.e.m. of 6 animals/group. (b) Oil Red O staining of WT and DKO brown preadipocyte cells differentiated for 8 days in the presence or in the absence of the thiazolidinedione roziglitasone (1 μM) or bone morphogenetic protein 7 (10 nM). A bright field microscopy picture of the differentiated cells is also shown. Scale bar=100 μm (c) Protein levels measured by western blot in WT and DKO cells before or 2, 4 and 8 days after induction of the differentiation. One representative blot from 3 independent experiments is shown. (d) mRNA abundance was measured by real time PCR in WT and DKO cells during the differentiation process before or 2, 4 and 8 days after induction of the differentiation. Results are mean±s.e.m. of 4 independent experiments. (e) Protein levels measured by western blot in WT and DKO cells during the first 3 days of differentiation. One representative blot from 3 independent experiments is shown. (f) Phosphorylation of C/EBPβ on Thr188, and C/EBPβ and δ levels were measured in WT and DKO cells in cytoplasmic and nuclear extracts, both in basal conditions and 4 h after the start of adipogenic conversion. One representative blot from 3 independent experiments is shown. Statistical significance assessed by two-tailed Student'st-test, *P<0.05. Figure 6: Adipocyte differentiation is impaired in DKO brown preadipocytes. ( a ) aP2, PPARγ, C/EBP α and C/EBP β mRNA abundance was measured by real time PCR in BAT from control and FIGIRKO male mice fed either a chow or a HFD. Results are mean±s.e.m. of 6 animals/group. ( b ) Oil Red O staining of WT and DKO brown preadipocyte cells differentiated for 8 days in the presence or in the absence of the thiazolidinedione roziglitasone (1 μM) or bone morphogenetic protein 7 (10 nM). A bright field microscopy picture of the differentiated cells is also shown. Scale bar=100 μm ( c ) Protein levels measured by western blot in WT and DKO cells before or 2, 4 and 8 days after induction of the differentiation. One representative blot from 3 independent experiments is shown. ( d ) mRNA abundance was measured by real time PCR in WT and DKO cells during the differentiation process before or 2, 4 and 8 days after induction of the differentiation. Results are mean±s.e.m. of 4 independent experiments. ( e ) Protein levels measured by western blot in WT and DKO cells during the first 3 days of differentiation. One representative blot from 3 independent experiments is shown. ( f ) Phosphorylation of C/EBPβ on Thr188, and C/EBPβ and δ levels were measured in WT and DKO cells in cytoplasmic and nuclear extracts, both in basal conditions and 4 h after the start of adipogenic conversion. One representative blot from 3 independent experiments is shown. Statistical significance assessed by two-tailed Student's t -test, * P <0.05. Full size image To better understand the reduction in adipose tissue mass and expression of key differentiation factors in FIGIRKO fat, we investigated the effect of knockout of the IR and IGF1R genes in brown preadipocytes in vitro [16] . Eight days after induction of differentiation, wild-type (WT) cells accumulated abundant lipid droplets that stained with Oil Red O ( Fig. 6b ). By contrast, no lipid accumulation was apparent in the IR and IGF1R double knockout (DKO) cells, indicating that insulin/IGF-1 signalling is critical for adipocyte differentiation. Addition of either the PPARγ agonist rosiglitazone or the brown adipogenesis inducer BMP-7 (ref. 17 ) were unable to rescue the lack of differentiation observed in DKO cells. This difference in adipocyte differentiation was also apparent in measurement of expression of adipocyte markers, which increased progressively at the mRNA and protein level in WT cells, but failed to be induced in DKO cells ( Fig. 6c,d ). As expected, PPARγ and C/EBPα mRNAs both increased by >20-fold in WT cells during adipocyte differentiation. By contrast, PPARγ and C/EBPα did not increase in DKO cells, indicating that insulin/IGF-1 signalling acts upstream of C/EBPα and PPARγ to induce adipocyte differentiation ( Fig. 6d ), most likely on C/EBPβ and C/EBPδ (refs [18] , [19] 18,19). C/EBPβ and C/EBPδ mRNA increased 20-fold rapidly after induction of differentiation both in WT and DKO cells ( Supplementary Fig. S7 ). This was confirmed at the protein level ( Fig. 6e ). However, C/EBPβ phosphorylation at threonine 188, which leads to DNA binding and transactivation of C/EBPα and PPARγ genes [20] , [21] , was significantly reduced in DKO cells, both under basal conditions and after addition of the induction cocktail ( Fig. 6f ). However, cellular localization of C/EBPβ and δ was normal in DKO cells compared with WT cells. Thus, insulin and IGF-1 signalling have a critical role in adipocyte differentiation, controlling C/EBPβ phosphorylation and activation upstream of C/EBPα and PPARγ. Impaired thermogenesis in FIGIRKO mice Although BAT is involved in thermogenesis, basal body temperature was similar between control and FIGIRKO mice ( Supplementary Fig. S8a ) raised at ~21 °C. However, when put in a 4°C environment, FIGIRKO mice were unable to maintain their body temperature. Thus, whereas control mice dropped their body temperature by only 3.5 °C after 90 min under these conditions, FIGIRKO mice dropped their body temperature by 12.6 °C, and all FIGIRKO mice had to be removed from the cold before 2 h owing to a drop of their body temperature below 25 °C ( Fig. 7a ). By contrast, mice with a fat-specific insulin receptor KO (FIRKO mice) that have a 50% reduction in BAT mass [14] and mice with a fat-specific knockout of the IGF1R that have normal BAT mass showed normal thermoregulation at 4 °C ( Supplementary Fig. S8b,c ). This defect was due to the major reduction in BAT mass in FIGIRKO mice, as well as a decrease in expression of genes involved in thermogenesis and various BAT markers. Thus, BAT from FIGIRKO mice had a 40% decrease in UCP1 mRNA levels compared with control ( Fig. 7b ), and this was paralleled by 41–75% decreases in PGC1α, PRDM16, Tfam, Nrf1, UCP3 and beta-adrenergic receptors Adrb1, 2 and 3 ( Fig. 7c ; Supplementary Fig. S8d ). Interestingly, expression of other BAT markers, such as Dio2, Elovl3 and Cox2, was not changed in BAT from FIGIRKO mice compared with control ( Supplementary Fig. S8d ), indicating that BAT from FIGIRKO mice has some alterations in differentiated function, but not a complete failure of differentiation. 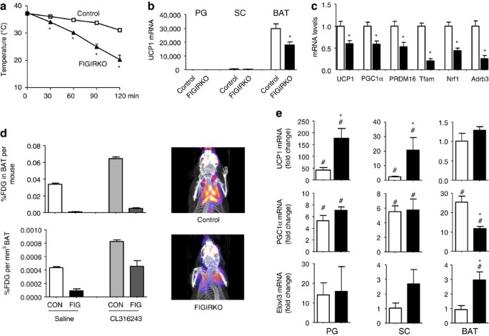Figure 7: FIGIRKO mice are extremely cold sensitive. (a) Rectal temperature was measured in 4 month old control and FIGIRKO male mice every 30 min for 2 h after exposure to a 4 °C environment (n=9 per group). (b)UCP1mRNA abundance was measured by real-time PCR in PG, SC and BAT in 4 month old male control and FIGIRKO mice. (c) mRNA abundance was measured by real-time PCR in BAT from 4 month old control and FIGIRKO male mice. Results are mean±s.e.m. of 6 animals/group. (d) Control and FIGIRKO mice were anesthetized and injected with 18-FDG. One hour after FDG injection, whole body PET-CT scans were performed and the interscapular area was analysed to measure FDG uptake in BAT. The experiment was repeated 1 h after injection of CL316243 (1 μg/g body weight) intraperitoneally. Results are mean±s.e.m. of 2 animals/group. Right panel show three-dimensional reconstruction images of control and FIGIRKO mice after FDG injection in the basal state. (e)UCP1, PGC1α andElovl3mRNA abundance was measured by real time PCR in PG, SC and BAT in 4 month old control and FIGIRKO male mice injected with either saline or CL316243 (1 μg/g body weight) intraperitoneally. Results are mean±s.e.m. of 5 animals/group and are expressed as fold change over the saline group. Statistical significance assessed by two-tailed Student'st-test, *P<0.05 between control and FIGIRKO mice, #P<0.05 between saline and CL316243 treated group. Figure 7: FIGIRKO mice are extremely cold sensitive. ( a ) Rectal temperature was measured in 4 month old control and FIGIRKO male mice every 30 min for 2 h after exposure to a 4 °C environment ( n =9 per group). ( b ) UCP1 mRNA abundance was measured by real-time PCR in PG, SC and BAT in 4 month old male control and FIGIRKO mice. ( c ) mRNA abundance was measured by real-time PCR in BAT from 4 month old control and FIGIRKO male mice. Results are mean±s.e.m. of 6 animals/group. ( d ) Control and FIGIRKO mice were anesthetized and injected with 18-FDG. One hour after FDG injection, whole body PET-CT scans were performed and the interscapular area was analysed to measure FDG uptake in BAT. The experiment was repeated 1 h after injection of CL316243 (1 μg/g body weight) intraperitoneally. Results are mean±s.e.m. of 2 animals/group. Right panel show three-dimensional reconstruction images of control and FIGIRKO mice after FDG injection in the basal state. ( e ) UCP1, PGC1 α and Elovl3 mRNA abundance was measured by real time PCR in PG, SC and BAT in 4 month old control and FIGIRKO male mice injected with either saline or CL316243 (1 μg/g body weight) intraperitoneally. Results are mean±s.e.m. of 5 animals/group and are expressed as fold change over the saline group. Statistical significance assessed by two-tailed Student's t -test, * P <0.05 between control and FIGIRKO mice, # P <0.05 between saline and CL316243 treated group. Full size image To determine BAT activity and its activation by β-adrenergic stimulation in vivo , we performed 18 F-fluorodeoxyglucose (FDG) positron-emission tomographic and computed tomographic (PET/CT) scans in control and FIGIRKO mice before and after intraperitoneal injection of the selective β3 adrenergic receptor agonist CL316243. Under basal conditions, FDG uptake was five times higher in BAT from control mice compared with FIGIRKO mice ( Fig. 7d ). One hour after CL316243 injection, FDG uptake increased 1.9-fold in BAT of control mice, and 5.2-fold in BAT from FIGIRKO mice, but uptake in FIGIRKO mice was still reduced by 45% compared with stimulated controls. When adjusted for the size differences in interscapular brown fat between the control and knockout mice, total FDG uptake was 35 and 13 times higher in BAT from control mice compared with FIGIRKO mice under basal and CL316243-activated conditions, respectively ( Fig. 7d ). Thus, BAT from FIGIRKO mice is dramatically reduced compared with BAT from control mice, but is still responsive to β3 adrenergic stimulation. We also measured gene expression in white and brown adipose tissues of mice injected with CL316243. After 3 h, UCP1 mRNA levels increased 45-fold and fourfold in PG and SC white adipose tissues of control mice, but not in BAT, probably because of the already extremely high UCP1 expression level in this tissue ( Fig. 7e ). In FIGIRKO mice, CL316243 induced an even greater increase in UCP1 with 175-fold and 20-fold increases in PG and SC, respectively. Similarly, CL316243 induced an increase in PGC1α and Elovl3 mRNA levels in adipose tissues of both control and FIGIRKO mice. These results indicate that absence of insulin and IGF-1 signalling in fat does not prevent the increased expression of genes involved in cold-induced thermogenesis. Thus, the cold sensitivity observed in FIGIRKO mice is likely due to the dramatic reduction in BAT mass and alteration in expression of key thermogenic genes, rather than an absence of induction of cold-induced stimulated genes. However, other potential mechanisms for the cold sensitivity such as decreased free fatty acid supply, decreased skeletal muscle ability to shiver or impaired heart or lung function cannot be excluded. Systemic brown adipocytes differ from the discrete or preformed interscapular BAT depot in their developmental origin [22] , [23] . They are found mixed in white fat and between muscle bundles [24] , arise from different progenitors than the cells giving rise to the preformed BAT, and are inducible by β3-adrenergic receptor stimulation and cold exposure. Daily injections of CL316243 for 2 weeks led to formation of systemic brown adipocytes within PG and SC white adipose tissue in control mice, as indicated by the increase in brown fat markers, histology and UCP1-immunostaining of fat from treated mice ( Supplementary Fig. S9a,b ). Interestingly, FIGIRKO mice also accumulated newly formed brown adipocytes in PG and SC adipose tissue depots to a similar extent than in control mice, indicating that while insulin/IGF-1 signalling is essential for preformed BAT formation, this pathway seems to be less important in the differentiation of systemic brown fat. Insulin and IGF-1 act through highly homologous receptors to initiate their functions on metabolism and growth. Although insulin and IGF-1 can have distinct physiological roles, at the cellular level, they regulate many of the same signalling pathways. We have previously shown that the IR and IGFR have similar effects in regulating gene expression in preadipocytes, with the main difference between insulin and IGF-1 effects being due to a modulation in amplitude of the signal created by the specific ligand–receptor interaction [12] . To understand the role of complementary actions of insulin and IGF-1 in fat metabolism and development, we created mice with a combined knockout of IR and IGFR in fat using Cre recombinase under the control of the adipocyte-specific aP2 promoter. The resulting FIGIRKO mice exhibit reduced body weight, reduced white adipocyte number, and an almost complete absence of BAT with dramatic sensitivity to cold exposure. Nonetheless, these mice are completely protected from age- and HFD-induced obesity and glucose intolerance, at least in part, owing to increased energy expenditure and increased glucose uptake in skeletal muscle. From the data, it seems that these changes occurred with only a partial knockdown of IR and IGF1R, because the mRNA levels of these two receptors in different fat depots were reduced only 30 to 60% in FIGIRKO mice. However, this is almost certainly an underestimate of the efficiency of the knockout, as inactivation of both IR and IGF1R dramatically impairs adipocyte differentiation, and in vivo , we can only assess the degree of inactivation in the residual adipose tissue in which the cells may have recombined some, but not all four, targeted alleles. This marked impairment of adipose tissue development, with some escaping cells, is consistent with the reduced number of normal-sized adipocytes observed in adipose tissues from FIGIRKO mice and is more than sufficient to produce a strong whole-body phenotype. The phenotype of the FIGIRKO mice differs drastically from that of mice with a fat-specific knockout of the insulin receptor (FIRKO). Whereas both mice have reduced white fat mass, this change is much greater in FIGIRKO mice, where there is a decrease in cell number compared with FIRKO mice, where there is primarily a change in cell size. Both FIRKO and FIGIRKO mice are protected against age-associated glucose intolerance and diet-induced obesity and glucose intolerance, and both display increased energy expenditure [14] , [25] . On the other hand, FIGIRKO mice are extremely cold sensitive and unable to exhibit an adequate thermogenic response when placed in the cold, whereas FIRKO mice show normal temperature regulation, indicating that the combined inactivation of the IR and IGF1R mediates some additional effects from that of IR alone on BAT development and function. These additional effects of the IGF1R are only observed when combined with a deletion of the IR. Thus, mice with adipocyte-specific deletion of IGF1R only have normal BAT mass, normal temperature regulation, and even an increase in white adipose tissue mass. The latter is part of a generalized increase in somatic growth, which has been attributed to increased circulating IGF-1 in these mice [15] . However, FIGIRKO mice have normal IGF-1 levels. The reduction in both white and brown adipocyte numbers in FIGIRKO mice reflects the important and synergistic roles of insulin and IGF-1 on the control of white and brown adipocyte differentiation. Both white and brown adipose tissues from FIGIRKO mice show reductions in adipocyte differentiation markers. Furthermore, IR and IGF1R double-knockout brown preadipocytes (DKO) fail to accumulate lipids or increase expression of adipocyte markers after induction of differentiation. C/EBPβ phosphorylation was strongly reduced in DKO cells, both under basal conditions or after induction of differentiation, indicating that insulin and IGF-1 signalling have a critical role in the control of adipocyte differentiation via activation and phosphorylation of C/EBPβ leading to impaired induction of C/EBPα and PPARγ. Interestingly, while insulin and IGF-1 signalling are essential for adipose development in the preformed, discrete BAT depots, they may not be required for differentiation of systemic brown adipocytes. These differences may be due to the differential lineages of these different brown fat depots [22] , [23] . This is also suggested by different molecular responses of precursors from these depots to a stimulation by a PPARγ agonist [26] . It is also possible that this pool of brown preadipocytes has a low level of aP2 expression compared with the preformed depot, limiting the extent of receptor inactivation in this population of cells. FIGIRKO mice are protected against age- and HFD-induced glucose intolerance. Interestingly, expression of inflammatory markers in adipose tissue and circulating cytokine levels are increased in FIGIRKO mice on high-fat diet to a similar level as in control mice, ruling out reduced inflammation in fat as a cause for the improved glucose tolerance observed in these mice. Improved glucose tolerance is also not due to differences in insulin secretion. However, insulin-stimulated glucose uptake is increased in skeletal muscle from FIGIRKO mice, and coupled with the increased insulin levels in HFD-fed FIGIRKO mice, it seems likely that the better glucose tolerance of FIGIRKO mice is due to increased insulin action in skeletal muscle. The most dramatic finding in FIGIRKO mice is the almost complete absence of interscapular BAT, highlighting the crucial role for insulin/IGF-1 signalling in BAT formation. BAT mass/activity in humans is inversely correlated with body mass index and percent body fat [2] , [3] , [4] , [27] , [28] , [29] . Interestingly, the defect in brown fat development in FIGIRKO mice is associated with increased energy expenditure and leanness. Although surprising, this is in agreement with the phenotype observed in UCP1-deficient mice which are cold sensitive [30] and protected from HFD-induced obesity when raised at 20 °C (ref. 31 ), but can become obese on HFD in a thermoneutral (29 °C) environment [32] . This suggests that for BAT to have a role in regulating energy expenditure, the tissue must have functional insulin and IGF-1 receptors. Exactly how FIGIRKO mice maintain temperature at 21 °C is unclear, as FIGIRKO mice do not show increased systemic brown adipocytes or increased expression of any UCP in the muscle, fat or the liver. Nevertheless, at 4 °C FIGIRKO mice are unable to maintain their body temperature, indicating that brown fat is essential for adaptative thermogenesis, similar to what has been observed in mice with UCP1 inactivation [30] . However, UCP1-deficient mice can be kept at 4 °C, if they are gradually adapted to the cold [33] , [34] , but this is because of shivering rather than the development of BAT-related thermogenesis [33] , [35] . Cold-induced thermogenesis is mediated via the sympathetic nervous system through activation of β-adrenergic receptors [36] , [37] . Despite the small BAT mass, the increase in FDG uptake after β3 stimulation is greater in FIGIRKO mice than controls. Furthermore, the β3 adrenergic agonist induced UCP1, PGC1α and Elovl3 expression in white and brown adipose tissues from both control and FIGIRKO mice to the same extent. However, the relative amount of FDG uptake is still lower in BAT from FIGIRKO mice in both basal and stimulated conditions indicating that in addition to the reduced BAT mass, BAT from FIGIRKO mice is less active. Taken together, these results highlight the critical role of insulin and IGF-1 signalling in the control of white and brown adipose tissue development and function, as well as the regulation of glucose metabolism and energy expenditure. Animals and diets Mice were housed in a temperature-controlled (20–22 °C) room on a 12 h-light/dark cycle in an animal facility at the Foster Biomedical Research Laboratory of Brandeis University in Waltham, MA, USA. All protocols were approved by the Institutional Animal Care and Use Committee of the Joslin Diabetes Center and Brandeis University and were in accordance with NIH guidelines. Mice were allowed ad libitum access to water and food. aP2-Cre from the Barbara Kahn laboratory and double IR and IGF1R floxed animals have been described previously [38] , [39] . Control and fat-specific IR and IGF1R KO (FIGIRKO) mice were maintained on a mixed (C57Bl/6 – 129Sv) background by breeding aP2-Cre IR f/f /IGF1R f/f with IR f/f /IGF1R f/f mice. Animals were maintained on a standard chow diet containing 22% calories from fat, 23% from protein, and 55% from carbohydrates (Mouse Diet 9F 5020; PharmaServ), or subjected to a HFD containing 60% calories from fat, 20% from protein, and 20% from carbohydrates (OpenSource Diet D12492, Research Diets). FIRKO mice and fat-specific IGF-1 receptor knockout mice (IGF-1RaP2Cre) have been described previously [14] , [15] . Adipocyte cell size Adipocytes from perigonadal and subcutaneous adipose tissue depots were dissected, minced and digested with 1 mg ml −1 collagenase I (Worthington Biosciences) in DMEM high glucose supplemented with 1% bovine serum albumin (BSA), shaking for 30 min at 37 °C. Cells were passed through a 200-μM filter and washed twice with DMEM high glucose plus BSA. Cells were fixed with osmium tetroxide, rinsed twice with PBS, and aliquots were used to take pictures on microscope slides. Adipocyte diameter from cells bigger than 20 μM was determined using Image J software. At least 5 pictures representing a total of ~1,000 per adipose tissue depot were used. 4 control and 4 FIGIRKO mice were used, representing a total of ~5,000 adipocytes per group. For brown adipocyte cell size, the number of cells/nuclei was determined from hematoxylin and eosin-stained sections of BAT from 4 FIGIRKO and 4 control mice. Average diameter of cells was determined for each slide. Metabolic studies Glucose tolerance and glucose stimulated insulin secretion tests (2 g dextrose per kg body weight, injected intraperitoneally) were performed in unrestrained conscious mice after a 16-h overnight fast. Insulin tolerance tests (1.25 units insulin per kg body weight injected intraperitoneally, Humulin R, Lilly) were performed after a 2 h fast. Glucose levels were measured in blood collected from the tail at the indicated times after injection, with Infinity glucose monitors and strips (US Diagnostics). Insulin sensitivity was directly and more precisely assessed by performing hyperinsulinemic–euglycemic clamps in conscious mice as described previously [40] , with a continuous insulin infusion dose of 2.5 mU kg −1 min −1 . Tissue triglyceride analysis Lipids from liver samples were extracted with Folch solution consisting of a mixture of 2:1 (v/v) chloroform/ methanol. Lipids were solubilized in 1% Triton X-100 and dried by evaporation. Triglyceride content was determined using Triglyceride Determination Kit (Sigma). Energy expenditure and body composition For the energy expenditure studies, 12 control and 12 FIGIRKO male mice were shipped to the Vanderbilt Mouse Metabolic Phenotyping Center. Oxygen consumption (VO 2 ), carbon dioxide (VCO 2 ) and heat production were measured by indirect calorimetry using the Comprehensive Laboratory Animal Monitoring System (Columbus Instruments) in 6-month old animals fed a chow diet. The respiratory exchange ratio (VCO 2 /VO 2 ) was calculated from the gas exchange data and all data were normalized to lean body mass. Half of the animals were then placed on a HFD for 4 months while the others remained on a chow diet, and body composition was assessed weekly by nuclear magnetic resonance. VO 2 , VCO 2 and heat production were measured again at the end of the diet. Body temperature and cold exposure Body temperatures were assessed in 4-month-old mice using a RET-3 rectal probe for mice (Physitemp). For the cold exposure experiment, mice were housed individually and transferred to a cold room with an ambient temperature of 4 °C. Temperature was measured every 30 min for 3 h, or until mouse core body temperature dropped below 25° C. In vivo BAT Imaging by PET/CT Mice were anaesthetized by intraperitoneal injection of pentobarbital at 75 mg kg −1 . Ten minutes post-injection of anaesthetic, saline or CL316243 was injected intraperitoneally at 1 mg kg −1 . Five minutes post-injection of drug, mice were then injected retro-orbitally with F18-FDG at 200–300 μCi. Time and exact amount of injected isotope was noted immediately after injection. Two hours post-injection of 18 F-FDG, mice were imaged by PET/CT on a NanoPET/CT (Bioscan) dual modality small animal imager. Thirty minutes before PET acquisition, all mice were given a subsequent dose of pentobarbital at 75 mg kg −1 to ensure adequate anaesthetization throughout the duration of the PET/CT scan. Gene expression analysis Total RNA was extracted from tissues with Trizol. RNA (1 μg) was reverse-transcribed with a high-capacity complementary DNA (cDNA) reverse transcription kit (Applied Biosystems) according to the manufacturer's instructions. Real-time PCR was performed starting with 12.5 ng of cDNA and both sense and antisense oligonucleotides (300 nM each) in a final volume of 10 μl with the SYBR Green PCR Master Mix (Applied Biosystems). Fluorescence was monitored and analysed in an ABI Prism 7900 HT sequence detection system (Applied Biosystems). Analysis of TATA box–binding protein expression was performed in parallel to normalize gene expression. Amplification of specific transcripts was confirmed by analysing melting curve profiles at the end of each PCR. Real-time PCR primers sequences are listed in Supplementary Table S1 . Cell culture and adipocyte differentiation DKO brown preadipocyte cell lines were generated from immortalized IR and IGF1R floxed brown preadipocytes infected with an adenovirus encoding Cre recombinase, as described previously [16] . Cells were maintained in DMEM (high glucose) containing 10% (v/v) fetal calf serum at 37 °C in a 5% CO 2 environment. Adipocyte differentiation was induced in confluent WT or DKO preadipocytes by treating confluent cells (day 0) with an induction mixture containing 20 nM insulin and 1 nM triiodothyronine, 0.5 mM isobutylmethylxanthine, 1 μM dexamethasone, and 0.125 mM indomethacin for 48 h. After this induction phase (day 2), cells were kept in medium containing insulin and triiodothyronine for the subsequent 6 days, changing the medium every 2 days. Lipid accumulation was visualized at day 8 by oil red O staining. Cells were washed once with phosphate-buffered saline and fixed with 10% buffered formalin for 1 h. Cells were then stained with filtered oil red O solution (5 g per liter in isopropyl alcohol) diluted twofold in water for 1 h at room temperature. Western blot analysis Cells were washed once with cold PBS and scraped in radioimmunoprecipitation assay lysis buffer containing 1% SDS, 10 mM glycerophosphate, 10 mM NaF, 0.1 mM. sodium orthovanadate, and 1% protease inhibitor cocktail (Sigma). For cytoplasmic and nuclear extracts, NE-PER Nuclear and Cytoplasmic Extraction Reagents (Thermo Scientific) were used according to manufacturer's instructions. Protein concentrations were determined with the Bradford protein assay (Bio-Rad). Lysates (20 to 40 μg) were subjected to SDS–polyacrylamide gel electrophoresis (SDS–PAGE). Proteins were transferred to a polyvinylidene difluoride membrane (Amersham Biosciences) and immunoblotted with the appropriate antibodies. Secondary antibodies were horseradish peroxidase (HRP)-conjugated anti-rabbit immunoglobulin G (IgG) from donkey and HRP-conjugated anti-mouse IgG from sheep (Amersham). Proteins on the membranes were visualized with SuperSignal West Pico substrate or SuperSignal West Dura extended-duration substrate (Pierce Biotechnologies). Antibodies (with catalogue number) to C/EBPα (sc-61), C/EBPβ (sc-150), C/EBPδ (sc-151), GLUT4 (sc-7938) and UCP1 (sc-6528) were purchased from Santa Cruz Biotechnologies (dilution 1/200). Antibodies to Phospho-C/EBPbeta (Thr188) (#3084) and Lamin A/C (#2032) were purchased from Cell Signaling (dilution 1/1,000). FAS (ab22759) and Superoxide dismutase 4 (ab16834) were purchased from Abcam (dilution 1/1,000). PPARγ (07-466) was purchased from Millipore (dilution 1/1,000). How to cite this article: Boucher, J. et al . Impaired thermogenesis and adipose tissue development in mice with fat-specific disruption of insulin and IGF-1 signalling. Nat. Commun. 3:902 doi: 10.1038/ncomms1905 (2012).